Synthetic quorum-sensing circuit to control consortial biofilm formation and dispersal in a microfluidic device To utilize biofilms for chemical transformations in biorefineries they need to be controlled and replaced. Previously, we engineered the global regulator Hha and cyclic diguanylate-binding BdcA to create proteins that enable biofilm dispersal. Here we report a biofilm circuit that utilizes these two dispersal proteins along with a population-driven quorum-sensing switch. With this synthetic circuit, in a novel microfluidic device, we form an initial colonizer biofilm, introduce a second cell type (dispersers) into this existing biofilm, form a robust dual-species biofilm and displace the initial colonizer cells in the biofilm with an extracellular signal from the disperser cells. We also remove the disperser biofilm with a chemically induced switch, and the consortial population could tune. Therefore, for the first time, cells have been engineered that are able to displace an existing biofilm and then be removed on command allowing one to control consortial biofilm formation for various applications. Biofilms are groups of cells at an interface cemented together by polysaccharides, protein, DNA and lipids [1] . Biofilms are related to most bacterial chronic inflammatory and infectious diseases [2] as well as involved in biocorrosion [3] and biofouling [4] in diverse areas. They also may be used for beneficial applications such as bioremediation and hold much potential for chemical transformations in biorefineries [5] . For these applications, compared with monocultures, mixed populations have the advantage of being able to perform more complex transformations (for example, those requiring multiple steps), and they are more resistant to environmental stress [6] . For these reasons, consortia have been heralded as the new frontier in synthetic biology [6] . However, to date, it has not been possible to control consortial biofilm formation. Based on an understanding of signals and regulatory networks during biofilm development [7] , biofilms have been engineered by manipulating extracellular/intercellular signals and regulators [5] . The first engineered biofilm was a consortium where Bacillus subtilis was engineered to secrete the peptide antimicrobials indolicidin and bactenecin to inhibit the growth of sulfate-reducing bacteria and thereby decrease corrosion [8] . Also, the first synthetic signalling circuit to control biofilm formation was developed for Escherichia coli and Pseudomonas fluorescens by manipulating the extracellular concentration of the signal indole produced by E. coli [9] ; indole is a biofilm inhibitor for E. coli . In addition, using directed evolution, the quorum-sensing (QS) regulator SdiA was reconfigured to decrease biofilm formation by increasing indole [10] , and the global regulator H-NS was evolved to decrease biofilm formation via prophage excision and cell death [11] . To remove existing biofilms, T7 bacteriophage was engineered to produce dispersin B of Actinobacillus actinomycetemcomitans to disrupt the glycosidic linkages of polymeric β-1,6- N -acetyl- D -glucosamine found in the biofilm matrix during bacteriophage infection [12] . In addition, the global transcriptional regulator Hha of E. coli , which reduces hemolysin production [13] and decreases biofilm formation [14] , was engineered using protein engineering (aa changes D22V, L40R, V42I and D48A) to enhance biofilm dispersal primarily by inducing protease HslV and cell lysis [15] , and BdcA, which increases biofilm dispersal by decreasing the concentration of the second messenger cyclic diguanylate (c-di-GMP) by binding it, was engineered (aa change E50Q) for nearly complete dispersal of biofilms [16] . Therefore, new genetic modules are available for manipulating biofilms [5] . Synthetic biology is an emerging field to develop biological systems that perform novel functions by assembling genetic modules [17] . The genetic modules include switches, cascades, pulse generators, time-delayed circuits, oscillators, spatial patterning and logic formulas, and they can be utilized to control transcription, translation and post-translational operations in order to tune gene expression, protein production, metabolism and cell–cell communication [18] . Among these genetic modules, bacterial QS systems are becoming important components of a wide variety of engineered biological devices [19] , as autoinducers are useful as input signals because most are small, diffuse freely in aqueous media and are easily imported by cells [20] . As the engineered cells synthesize their own QS signals, they are able to monitor their cell density and modulate their activities [21] accordingly without supervision. Hence, QS-based circuits have a wide range of potential engineering applications such as production of biochemicals, tissue engineering and mixed-species fermentations as well as developing biosensors and controlling biofouling [20] . For example, LuxI from Vibrio fischeri , which produces N -(3- oxo -hexanoyl)- L -homoserine lactone (3 o C6HSL) and AiiA from B. thuringiensis , which degrades 3 o C6HSL, were utilized to generate synchronized oscillations [22] . Also, the LuxI/LuxR QS system was coupled to the production of a toxin protein CcdB to induce cell death at high cell densities [23] , and applied to create programmable cell behaviour that synthesizes a target protein when the cell population reaches a critical density [24] . The two best-characterized QS systems of P. aeruginosa are the LasI/LasR and RhlI/RhlR systems, which regulate biofilm formation, virulence, swarming motility and antibiotic efflux pumps [25] . LasI produces autoinducer molecule, N -(3- oxo -dodecanoyl)- L -homoserine lactone (3 o C12HSL), which is sensed by LasR [26] . Likewise, RhlI produces N -butyryl- L -homoserine lactone (C4HSL) that is sensed by RhlR [26] . The LasI/LasR and RhlI/RhlR QS systems have been used to engineer bidirectional communication [27] , and the LasI/LasR QS system was used to both construct a predator–prey ecosystem [28] and create a synthetic ecosystem in E. coli [29] . Furthermore, the RhlI/RhlR QS system was utilized to demonstrate roles for self-organization and aggregation in a synthetic biofilm consortium [30] . Hence, synthetic QS circuit systems have potential in that population-driven QS switches may be utilized to develop synthetic genetic networks for a variety of applications. As biofilm formation and dispersal are ultimately genetic processes, they may be manipulated like other genetic systems [5] using the tools of synthetic biology [18] and directed evolution. In this work, our goal was to control biofilm displacement via a population-driven QS switch coupled to engineered biofilm dispersal proteins. Controlling biofilm dispersal creates a synthetic biological platform for sophisticated patterning of biofilms for engineering applications. The LasI/LasR QS module of P. aeruginosa was combined with our engineered Hha [15] and BdcA [16] biofilm dispersal proteins, and the system was utilized to selectively remove one type of cell from an existing biofilm, and then remove the second biofilm to create a surface ready for additional biofilms. Constructs were also created that allow the consortial population to be tuned. Therefore, for the first time, a quorum sensing circuit has been devised that allows biofilm formation to be controlled to the extent each cell type may be dispersed allowing one to control consortial biofilm formation for various applications. Microfluidic biofilm engineering circuit The microfluidic biofilm engineering (μBE) signalling circuit was constructed in E. coli using two engineered biofilm-dispersing proteins, Hha13D6 (ref. 15 ) and BdcAE50Q [16] , along with the P. aeruginosa LasI/LasR QS system ( Fig. 1a ) for use in the novel microfluidic device ( Fig. 1b ). E. coli hha [31] was used as the host as deletion of hha increases biofilm formation [14] and provides a background in which there is no wild-type Hha. Lactococcal promoter CP25 [32] was used as the strong constitutive promoter for two of the three proteins on each plasmid. To obtain high concentrations of intercellular signal 3 o C12HSL and regulator LasR, a synthetic ribosomal-binding site (RBS II) [32] was first utilized. However, high expression of lasI or lasR was deleterious; thus, we used the native RBS of these genes. All the cloned genes for the two cell types were placed on a single plasmid (pCA24N derivative, Fig. 2a,b ) to avoid plasmid instability and so that a single antibiotic could be used to maintain the key plasmid during growth of the consortia. 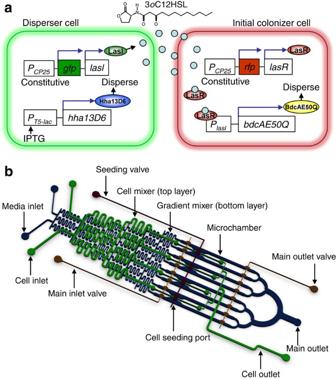Figure 1: μBE metabolic circuit and microfluidic device. (a) The twoE. colicell types communicate by using the LasI/LasR QS module ofP. aeruginosa. In the disperser cell, the LasI protein (autoinducer synthase) is constitutively produced and synthesizes the QS signal 3oC12HSL. 3oC12HSL freely diffuses into the initial colonizer cell and makes a complex with LasR (LuxR family transcriptional regulator), and the 3oC12HSL+LasR complex induces biofilm dispersal protein BdcAE50Q by activating thelasIpromoter. BdcAE50Q disperses biofilms by binding cyclic diguanylate. The biofilm dispersal protein Hha13D6 in the disperser cell is induced upon adding IPTG. Hha13D6 disperses biofilms by activating proteases. (b) The novel microfluidic device is shown with its two PDMS layers, a bottom layer with a diffusive mixer and eight microchambers, and a top layer containing a second diffusive mixer and the pneumatic elements to control microvalves. The diffusive mixer in the bottom layer was used to generate different concentrations of dispersal signals (for example, IPTG for removing disperser cells and 3oC12HSL for dispersing initial colonizer cells) and to perfuse growth media into the biofilm microchambers. The mixer in the top layer was used to introduce bacteria into the microchambers at different cell densities. Figure 1: μBE metabolic circuit and microfluidic device. ( a ) The two E. coli cell types communicate by using the LasI/LasR QS module of P. aeruginosa . In the disperser cell, the LasI protein (autoinducer synthase) is constitutively produced and synthesizes the QS signal 3 o C12HSL. 3 o C12HSL freely diffuses into the initial colonizer cell and makes a complex with LasR (LuxR family transcriptional regulator), and the 3 o C12HSL+LasR complex induces biofilm dispersal protein BdcAE50Q by activating the lasI promoter. BdcAE50Q disperses biofilms by binding cyclic diguanylate. The biofilm dispersal protein Hha13D6 in the disperser cell is induced upon adding IPTG. Hha13D6 disperses biofilms by activating proteases. ( b ) The novel microfluidic device is shown with its two PDMS layers, a bottom layer with a diffusive mixer and eight microchambers, and a top layer containing a second diffusive mixer and the pneumatic elements to control microvalves. The diffusive mixer in the bottom layer was used to generate different concentrations of dispersal signals (for example, IPTG for removing disperser cells and 3 o C12HSL for dispersing initial colonizer cells) and to perfuse growth media into the biofilm microchambers. The mixer in the top layer was used to introduce bacteria into the microchambers at different cell densities. 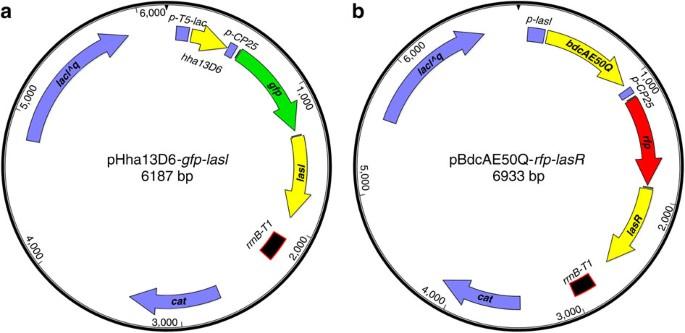Figure 2: Plasmid maps of the disperser plasmid and the initial colonizer plasmid that are used to create the μBE circuit. (a) pHha13D6-gfp-lasIwithhha13D6under control of theT5-lacpromoter, andgfpandlasIunder control of the constitutive CP25 promoter. (b) pBdcAE50Q-rfp-lasRwithbdcAE50Qunder control of thelasIpromoter, andrfpandlasRunder control of the constitutive CP25 promoter.catencodes chloramphenicol acetyltransferase,lacI^qencodes a repressor mutant of thelacoperator andrrnB-T1indicates therrnBT1 transcription termination sequence. Full size image Figure 2: Plasmid maps of the disperser plasmid and the initial colonizer plasmid that are used to create the μBE circuit. ( a ) pHha13D6- gfp - lasI with hha13D6 under control of the T5-lac promoter, and gfp and lasI under control of the constitutive CP25 promoter. ( b ) pBdcAE50Q- rfp - lasR with bdcAE50Q under control of the lasI promoter, and rfp and lasR under control of the constitutive CP25 promoter. cat encodes chloramphenicol acetyltransferase, lacI ^ q encodes a repressor mutant of the lac operator and rrnB-T1 indicates the rrnB T1 transcription termination sequence. Full size image In the μBE circuit, disperser cells ( lasI + , hha13D6 + , gfp + via E. coli hha/ pHha13D6- gfp - lasI ) produce constitutively green fluorescent protein (GFP) and the QS signal 3 o C12HSL, and have hha13D6 induced upon addition of isopropyl-β- D -thiogalactopyranoside (IPTG) ( Fig. 1a ). The initial colonizer cells ( lasR + , bdcAE50Q + , rfp + via E. coli hha/ pBdcAE50Q- rfp - lasR ) produce constitutively red fluorescent protein (RFP) and regulator LasR, the receptor of 3 o C12HSL. The initial colonizer cells also have bdcAE50Q under the control of the lasI promoter, which is activated via the 3 o C12HSL+LasR complex [33] ( Fig. 1a ). Thus, disperser cells produce the signalling molecule 3 o C12HSL, and the initial colonizer biofilm-forming cells sense it and disperse when the disperser cells reach a quorum. Disperser cells grow more slowly than the initial colonizer cells As we desire the disperser cells to supplant the initial colonizer cells, we checked the specific growth rates of the two strains to see if they are comparable; the disperser cells grew 14% slower than the initial colonizer cells in rich medium (Luria-Bertani (LB)-glucose, μ disperser =1.13±0.08 h −1 and μ initial colonizer =1.31±0.05 h −1 , respectively). The slower growth of the disperser cells is due to somewhat leaky expression of toxin hha13D6 rom the T5-lac promoter [34] , as a strain with a plasmid with the araBAD promoter to better repress hha13D6 in the absence of arabinose (pPBAD- hha13D6 - gfp - lasI ) increased the growth of the disperser cells by 12% ( μ disperser with araBAD promoter =1.27±0.23 h −1 ) ( Supplementary Methods ). Corroborating this difference in cell growth, disperser cells formed biofilms more slowly compared with initial colonizer cells: the biomass of initial colonizer cells after 9 h was 5.7±0.1 μm 3 μm −2 ( Fig. 3a ), while the biomass of the disperser cells after 9 h was 4.1±0.1 μm 3 μm −2 ( Fig. 3b ). 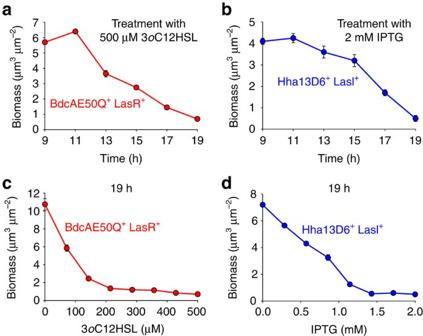Figure 3: Biomass of initial colonizer and disperser biofilms. (a) Biomass of initial colonizer biofilms (BdcAE50Q+and LasR+;E. coli hha/pBdcAE50Q-rfp-lasR) with 500 μM of 3oC12HSL for 10 h. (b) Biomass of disperser biofilms (Hha13D6+and LasI+;E. coli hha/pHha13D6-gfp-lasI) with 2 mM of IPTG for 10 h. (c) Biomass after 19 h for the initial colonizer biofilms with different concentrations of 3oC12HSL (0, 71, 143, 214, 286, 357, 429 and 500 μM for 10 h). (d) Biomass after 19 h for the disperser biofilms with different concentrations of IPTG (0, 0.3, 0.6, 0.9, 1.1, 1.4, 1.7 and 2.0 mM for 10 h). Robust biofilms at 9 h were formed by seeding the initial colonizer or the disperser cells into microchambers for (a), (b), (c) and (d). Three independent cultures were tested, and error bars indicate the s.d. from two different positions in one of the three sets. Biomass was determined by COMSTAT analysis. Figure 3: Biomass of initial colonizer and disperser biofilms. ( a ) Biomass of initial colonizer biofilms (BdcAE50Q + and LasR + ; E. coli hha/ pBdcAE50Q- rfp - lasR ) with 500 μM of 3 o C12HSL for 10 h. ( b ) Biomass of disperser biofilms (Hha13D6 + and LasI + ; E. coli hha/ pHha13D6- gfp - lasI ) with 2 mM of IPTG for 10 h. ( c ) Biomass after 19 h for the initial colonizer biofilms with different concentrations of 3 o C12HSL (0, 71, 143, 214, 286, 357, 429 and 500 μM for 10 h). ( d ) Biomass after 19 h for the disperser biofilms with different concentrations of IPTG (0, 0.3, 0.6, 0.9, 1.1, 1.4, 1.7 and 2.0 mM for 10 h). Robust biofilms at 9 h were formed by seeding the initial colonizer or the disperser cells into microchambers for ( a ), ( b ), ( c ) and ( d ). Three independent cultures were tested, and error bars indicate the s.d. from two different positions in one of the three sets. Biomass was determined by COMSTAT analysis. Full size image Disperser cells produce 3 o C12HSL To confirm the disperser μBE circuit synthesizes 3 o C12HSL, we measured the 3 o C12HSL concentration of the disperser cells ( E. coli hha/ pHha13D6- gfp - lasI ) in the biofilm using a lacZ reporter ( lasB – lacZ translational fusion) that is activated by 3 o C12HSL ( Supplementary Methods ) [35] . In flow cells, disperser cells in biofilms produced 14-fold higher concentrations of 3 o C12HSL compared with the planktonic cells in the effluent (6.7±2.1 μM versus 0.5±0.2 μM), and produced 51-fold higher concentrations of 3 o C12HSL compared with planktonic cells in shake flasks (0.1±0.1 μM). The negative control (no lasI ) had no detectable 3 o C12HSL. These results confirm that autoinducer concentrations in biofilms are higher than in planktonic cultures [36] and compare well with levels of 3 o C12HSL produced in P. aeruginosa biofilms (1 [37] –600 μM [36] ). As maximum activity of the lasI promoter is obtained with 0.1 μM of 3 o C12HSL and LasR [33] , 3 o C12HSL production in the disperser biofilms should induce the lasI promoter in the LasR-producing initial colonizer cells to express bdcAE50Q to disperse the initial colonizer biofilms. Moreover, as 3 o C12HSL diffusion is significantly slower compared with C4HSL diffusion [38] , local concentrations of 3 o C12HSL in biofilms may be much higher than the 3 o C12HSL concentration measured here. 3 o C12HSL disperses the initial colonizer biofilm To demonstrate that 3 o C12HSL disperses biofilms produced by the initial colonizer cells ( E. coli hha/ pBdcAE50Q- rfp - lasR ) by binding LasR and inducing bdcAE50Q , exogenous 3 o C12HSL at different concentrations was added to biofilms formed by the initial colonizer cells in microfluidic channels. As expected, the initial colonizer biofilms were dispersed upon adding 3 o C12HSL in a dose-dependent manner ( Fig. 3c ; Supplementary Fig. S1 ); near complete biofilm dispersal was obtained at 500 μM of 3 o C12HSL, and at lower 3 o C12HSL concentrations, dispersal of the initial colonizer biofilms was reduced ( Supplementary Fig. S1 ). In contrast, there was no dispersal in the absence of 3 o C12HSL ( Supplementary Fig. S1 ), and the initial colonizer cells formed thick biofilms (10.8±0.6 μm 3 μm −2 ) ( Fig. 3c ). Hence, initial colonizer cells recognize 3 o C12HSL and this signal may be used to disperse initial colonizer biofilms. IPTG removes the disperser biofilm To demonstrate that IPTG disperses biofilms produced by disperser cells by inducing hha13D6 , exogenous IPTG at different concentrations was added to biofilms formed by disperser cells in microfluidic channels. As expected, disperser biofilms were dispersed upon adding IPTG in a dose-dependent manner ( Fig. 3d ) with near complete biofilm dispersal at 2 mM IPTG ( Supplementary Fig. S2 ); hence, we used 2 mM IPTG in subsequent experiments. In contrast, there was no dispersal in the absence of IPTG ( Supplementary Fig. S2 ). Thus, the disperser cell has active hha13D6 to disperse its own biofilm upon IPTG addition. Engineered BdcA and Hha are necessary for biofilm dispersal To confirm that the biofilm dispersal upon addition of 3 o C12HSL and IPTG is the result of production of the engineered biofilm dispersal proteins, we performed dispersal experiments of initial colonizer cells that lack bdcAE50Q and disperser cells that lack hha13D6 . As expected, initial colonizer biofilms formed without bdcAE50Q (via E. coli hha/ pRFP- lasR ) did not disperse in the presence of 3 o C12HSL ( Fig. 4a ), while initial colonizer biofilms formed with bdcAE50Q dispersed with 3 o C12HSL ( Supplementary Fig. S1 ). Similarly, disperser biofilms formed without hha13D6 (via E. coli hha/ pGFP- lasI ) did not disperse upon addition of IPTG ( Fig. 4b ), while disperser biofilms formed with hha13D6 dispersed with IPTG ( Supplementary Fig. S2 ). Hence, BdcAE50Q and Hha13D6 are necessary to disperse the initial colonizer and disperser biofilms, respectively. Taken together, both disperser and initial colonizer cells were constructed to allow us to manipulate biofilm dispersal using a population-driven switch. 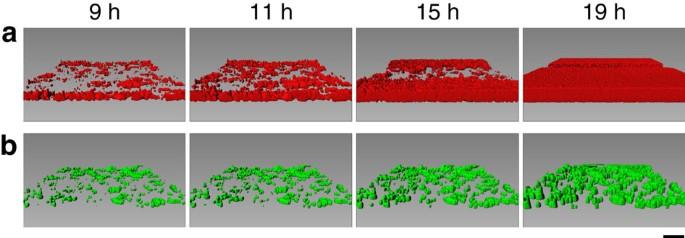Figure 4: Biofilms formed by cells that lack their respective biofilm dispersal proteins. (a) Initial colonizer biofilms that lack BdcA (BdcAE50Q−and LasR+viaE. coli hha/pRFP-lasR) with 500 μM of 3oC12HSL for 10 h. (b) Disperser biofilms that lack Hha (Hha13D6−and LasI+viaE. coli hha/pGFP-lasI) with 2 mM of IPTG for 10 h. Robust biofilms of initial colonizer or disperser cells were developed for 9 h in each microchamber. Scale bar indicates 20 μm. Three independent cultures were tested, and representative images are shown. Figure 4: Biofilms formed by cells that lack their respective biofilm dispersal proteins. ( a ) Initial colonizer biofilms that lack BdcA (BdcAE50Q − and LasR + via E. coli hha/ pRFP- lasR ) with 500 μM of 3 o C12HSL for 10 h. ( b ) Disperser biofilms that lack Hha (Hha13D6 − and LasI + via E. coli hha/ pGFP- lasI ) with 2 mM of IPTG for 10 h. Robust biofilms of initial colonizer or disperser cells were developed for 9 h in each microchamber. Scale bar indicates 20 μm. Three independent cultures were tested, and representative images are shown. Full size image Disperser cells displace initial colonizer biofilms Having verified the disperser and initial colonizer cell elements of the μBE signalling circuit, we combined both cell types to form a consortial biofilm and investigated whether the disperser cells could displace the initial colonizer cells. First, robust biofilms of initial colonizer cells were developed for 9 h after seeding, and then disperser cells were added to the initial colonizer biofilms for 5 h to form the biofilm consortium ( Fig. 5a ; Supplementary Movie 1 ). As disperser cells synthesize 3 o C12HSL constitutively, 3 o C12HSL should bind to LasR when the concentration of 3 o C12HSL is increased as the disperser biofilms mature. Then, the 3 o C12HSL+LasR complex should induce dispersal of initial colonizer biofilms by switching on bdcAE50Q under control of the lasI promoter. As expected, the initial colonizer biofilms were displaced from the surface as the disperser cells grew ( Fig. 5a ; Supplementary Movie 1 ). After 44 h, 80% of the maximum initial colonizer biofilm formed was removed ( Fig. 5a,b ; Supplementary Movie 1 ). The displacement of the initial colonizer cells by the disperser cells was accomplished by the production of 3 o C12HSL from the disperser biofilms, not by shear force, as the disperser biofilms that lack LasI did not reduce initial colonizer biofilms; that is, both no lasI disperser and initial colonizer biofilms grew when 3 o C12HSL was not produced ( Fig. 5c ), and the biofilm became essentially that of the faster-growing initial colonizer cells after 40 h ( Fig. 5c,d ). Hence, the disperser cells completely displaced the initial colonizer biofilm via the population-driven synthetic μBE system. 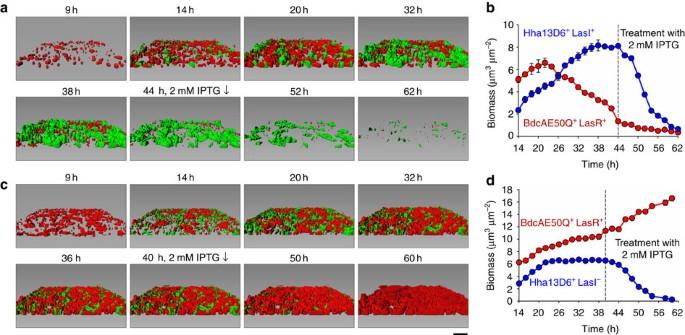Figure 5: Dispersal of dual-species biofilms using quorum sensing. (a) An initial colonizer biofilm (red, BdcAE50Q+and LasR+;E. coli hha/pBdcAE50Q-rfp-lasR) was developed for 9 h, then disperser cells (green, Hha13D6+and LasI+;E. coli hha/pHha13D6-gfp-lasI) were seeded for 5 h to form both initial colonizer and disperser biofilms. After 44 h, 2 mM of IPTG was added for an additional 18 h to remove the disperser biofilm. (b) Biomass of the initial colonizer (BdcAE50Q+and LasR+) and disperser (Hha13D6+and LasI+) biofilms as determined by COMSTAT analysis. (c) Initial colonizer biofilms (BdcAE50Q+and LasR+) was developed for 9 h, then control disperser cells that lack LasI (green, Hha13D6+and LasI−;E. coli hha/pHha13D6-gfp) were seeded for 5 h to form both initial colonizer and control disperser biofilms. After 40 h, 2 mM of IPTG was introduced for an additional 20 h to try to disperse the control disperser biofilms, which lacklasI. (d) Biomass of the initial colonizer (BdcAE50Q+and LasR+) and the no LasI disperser control (Hha13D6+and LasI−) biofilms as determined by COMSTAT analysis. Scale bar indicates 20 μm. Three independent cultures were tested, and representative images are shown for (a) and (c). Error bars indicate the s.d. from two different positions in one of the three sets for (b) and (d). Figure 5: Dispersal of dual-species biofilms using quorum sensing. ( a ) An initial colonizer biofilm (red, BdcAE50Q + and LasR + ; E. coli hha/ pBdcAE50Q- rfp - lasR ) was developed for 9 h, then disperser cells (green, Hha13D6 + and LasI + ; E. coli hha/ pHha13D6- gfp - lasI ) were seeded for 5 h to form both initial colonizer and disperser biofilms. After 44 h, 2 mM of IPTG was added for an additional 18 h to remove the disperser biofilm. ( b ) Biomass of the initial colonizer (BdcAE50Q + and LasR + ) and disperser (Hha13D6 + and LasI + ) biofilms as determined by COMSTAT analysis. ( c ) Initial colonizer biofilms (BdcAE50Q + and LasR + ) was developed for 9 h, then control disperser cells that lack LasI (green, Hha13D6 + and LasI − ; E. coli hha/ pHha13D6- gfp ) were seeded for 5 h to form both initial colonizer and control disperser biofilms. After 40 h, 2 mM of IPTG was introduced for an additional 20 h to try to disperse the control disperser biofilms, which lack lasI . ( d ) Biomass of the initial colonizer (BdcAE50Q + and LasR + ) and the no LasI disperser control (Hha13D6 + and LasI − ) biofilms as determined by COMSTAT analysis. Scale bar indicates 20 μm. Three independent cultures were tested, and representative images are shown for ( a ) and ( c ). Error bars indicate the s.d. from two different positions in one of the three sets for ( b ) and ( d ). Full size image The second key element of our design was the removal of the disperser biofilm; we found, we could remove the disperser biofilm by inducing Hha13D6 with IPTG ( Fig. 5a ). After 62 h (18 h with 2 mM IPTG), 92% of the maximum disperser biofilm was removed ( Fig. 5b ). Note that the 3 o C12HSL signal is still made while IPTG is added so the small number of remaining colonizer cells are not able to form a biofilm while the disperser cells are being removed. Fine-tuning consortial populations using the araBAD promoter To fine-tune the consortial composition, a plasmid with the araBAD promoter instead of the lasI promoter for bdcAE50Q was constructed so that BdcAE50Q may be produced in the initial colonizer cells by adding arabinose. We confirmed the activity of the araBAD promoter in the new construct by testing the swimming motility of the new colonizer strain ( E. coli hha /pPBAD- bdcAE50Q-rfp-lasR ), as BdcAE50Q decreases the concentration of c-di-GMP by binding it and thereby increases swimming motility ( Supplementary Methods ) [16] . As expected, swimming motility of the araBAD promoter-controlled initial colonizer strain was increased 2.2±0.3-fold by adding arabinose (halo diameter 6.2±0.1 cm with 0.2% arabinose versus 2.8±0.1 cm with no arabinose), whereas the swimming motility of the old initial colonizer strain ( E. coli hha /pBdcAE50Q -rfp-lasR ) was not changed by arabinose addition ( Supplementary Fig. S3 ). Hence, the araBAD promoter controls bdcAE50Q expression as a function of arabinose concentration. To disperse the new initial colonizer cells ( E. coli hha /pPBAD- bdcAE50Q - rfp - lasR , red, initial colonizer-2), we added arabinose (1 wt%) after both the initial colonizer-2 and the disperser biofilms were formed in the microfluidic channel. Dispersal of the initial colonizer-2 biofilm increased with production of BdcAE50Q via arabinose addition ( Fig. 6a,b ). Therefore, the initial colonizer-2 cells could be dispersed upon adding arabinose. 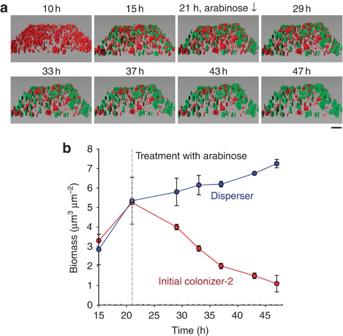Figure 6: Dispersal of dual-species biofilms using arabinose. (a) Initial colonizer-2 biofilms (E. coli hha/pPBAD-bdcAE50Q-rfp-lasR, red) were developed in the microfluidic device for 10 h, then disperser cells (E. coli hha/pHha13D6-gfp-lasI, green) were seeded for 5 h to form both initial colonizer-2 and disperser biofilms in LB-glucose medium. After 21 h, 1% arabinose in tryptone medium was added for an additional 26 h to disperse the initial colonizer-2 biofilm. Three independent cultures were tested, and representative images of biofilms from channel 2 at each time point are shown. Scale bar indicates 20 μm. (b) Biomass (μm3μm−2) of initial colonizer-2 and disperser biofilms at each time point in channel 2. Error bars indicate the s.d. from two different positions. Figure 6: Dispersal of dual-species biofilms using arabinose. ( a ) Initial colonizer-2 biofilms ( E. coli hha /pPBAD- bdcAE50Q - rfp - lasR , red) were developed in the microfluidic device for 10 h, then disperser cells ( E. coli hha/ pHha13D6- gfp - lasI , green) were seeded for 5 h to form both initial colonizer-2 and disperser biofilms in LB-glucose medium. After 21 h, 1% arabinose in tryptone medium was added for an additional 26 h to disperse the initial colonizer-2 biofilm. Three independent cultures were tested, and representative images of biofilms from channel 2 at each time point are shown. Scale bar indicates 20 μm. ( b ) Biomass (μm 3 μm −2 ) of initial colonizer-2 and disperser biofilms at each time point in channel 2. Error bars indicate the s.d. from two different positions. Full size image To vary the consortial biofilm population in the microfluidic device using the araBAD promoter and the initial colonizer-2 strain so that the population could be controlled by arabinose addition, a gradient of initial colonizer-2 biofilms was developed across the channels 1 through 8 of the microfluidic device. In this setup, the maximum initial colonizer-2 biofilm is formed in channel 8, then a uniform concentration of disperser cells ( E. coli hha/ pHha13D6- gfp - lasI , green) were seeded in all eight channels to form both initial colonizer-2 and disperser biofilms at different biofilm ratios across the eight channels at 21 h ( Fig. 7a ). The initial colonizer-2 biofilms were dispersed to various degrees from 62% dispersal in channel 2 to 26% dispersal in channel 6 at 37 h, while the disperser biofilms were not affected ( Fig. 7b ). Thus, the consortial population of initial colonizer and disperser cells may be controlled. 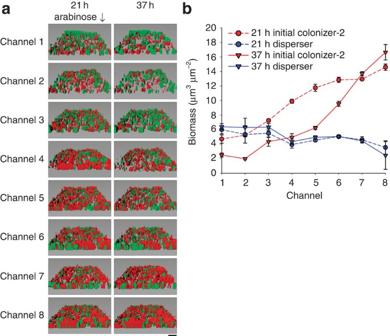Figure 7: Population dynamics of initial colonizer-2 and disperser biofilms. (a) A gradient of initial colonizer-2 biofilms (E. coli hha/pPBAD-bdcAE50Q-rfp-lasR, red) was developed across channels 1 through 8 in the microfluidic device for 10 h such that the maximum initial colonizer-2 biofilm was formed in channel 8, then a uniform concentration of disperser cells (E. coli hha/pHha13D6-gfp-lasI, green) were seeded for 5 h in all eight channels to form both initial colonizer-2 and disperser biofilms in LB-glucose medium at different biofilm ratios across the eight channels. After 21 h, 1% arabinose in tryptone medium was added to disperse the initial colonizer-2 biofilm. Three independent cultures were tested, and representative images of biofilms at time 21 h and 37 h are shown. Scale bar indicates 20 μm. (b) Biomass (μm3μm−2) of initial colonizer-2 and disperser biofilms at time 21 h and 37 h in the eight channels. Error bars indicate the s.d. from two different positions. Figure 7: Population dynamics of initial colonizer-2 and disperser biofilms. ( a ) A gradient of initial colonizer-2 biofilms ( E. coli hha /pPBAD- bdcAE50Q - rfp - lasR , red) was developed across channels 1 through 8 in the microfluidic device for 10 h such that the maximum initial colonizer-2 biofilm was formed in channel 8, then a uniform concentration of disperser cells ( E. coli hha/ pHha13D6- gfp - lasI , green) were seeded for 5 h in all eight channels to form both initial colonizer-2 and disperser biofilms in LB-glucose medium at different biofilm ratios across the eight channels. After 21 h, 1% arabinose in tryptone medium was added to disperse the initial colonizer-2 biofilm. Three independent cultures were tested, and representative images of biofilms at time 21 h and 37 h are shown. Scale bar indicates 20 μm. ( b ) Biomass (μm 3 μm −2 ) of initial colonizer-2 and disperser biofilms at time 21 h and 37 h in the eight channels. Error bars indicate the s.d. from two different positions. Full size image We developed a synthetic μBE system by combining a QS signalling module with two of our engineered biofilm dispersal proteins. With this synthetic circuit, in a microfluidic channel, we formed an initial colonizer biofilm with cells tagged red, introduced a second cell type (dispersers, tagged green) into this existing biofilm, created a means of communication between the two cell types and formed a robust biofilm with the disperser cells in an existing initial colonizer biofilm. We then displaced the initial colonizer cells in the biofilm with a QS signal from the disperser cells, and removed the disperser cells with a chemically induced switch. Our work demonstrates that biofilms can be formed, that new cells may be engineered to integrate and then replace the initial colonizer biofilm, and that both cell types may be removed, which is a promising strategy for applications requiring different kinds of engineered cells such as creating a biorefinery. Although some of the biofilms may be dispersed naturally upon changes in environmental conditions (for example, nutrition level and oxygen depletion) [39] , it is a significant challenge to remove biofilms [40] , [41] as cells in biofilms are cemented in place by the secreted polymer matrix consisting of polysaccharide, protein, DNA and lipids [1] . The matrix holds bacterial cells together and forms a protective barrier that confers resistance to killing by nonspecific and specific host defenses during infection and that confers tolerance to various antimicrobial agents such as disinfectants and antibiotics [1] . Thus, the defensive nature of the biofilm colony makes most biofilms difficult or impossible to eradicate [39] ; hence, our demonstration that both the initial colonizer and disperser biofilms may be nearly completely removed is significant. To preferentially remove one type of cell in a biofilm, our system requires that the second cell type elicits robust growth such that it can attach to the existing biofilm and propagate, that it flourishes, that it communicates to the other cell type via a QS signal, and that it displaces the existing biofilm without itself being displaced so that it instead forms a strong biofilm. Here, we produced the QS signal in the biofilm itself to remove the initial colonizer cells. As the signal accumulated, the engineered BdcA in the initial colonizer cells reduces c-di-GMP levels, which results in a cascade of events, such as an increase in motility and reduction in adhesion production, that allows the initial colonizer cells to disperse [16] . As the initial colonizer cells disperse, the disperser cells must form a robust biofilm. After the disperser biofilm is formed, the engineered Hha protein, once induced, causes dispersal by inducing cell lysis [15] . Therefore, our synthetic μBE system provides a useful platform for the removal of existing deleterious biofilms via generating signalling molecules in situ . In addition, as the disperser cells grow more slowly than the initial colonizer ones, the disperser cells cannot displace the initial colonizer biofilm based on a difference in growth rates. This clearly demonstrates that a QS circuit was required to complete this feat of progressive biofilm development/dispersal. As several biofilm dispersal signals have been identified including the auto-inducing peptide of the agr QS system of Staphylococcus aureus [42] , changes in carbon sources [43] , reduction in the concentration of c-di-GMP [16] (as utilized here with BdcA), surfactant [44] , cis -2-decenoic acid [45] , as well as D -amino acids [46] , we envision that other biofilm dispersal mechanisms may also be utilized to control biofilms. The μBE device described here offers several advantages over the commercially available BioFlux device developed by Benoit et al . [47] and other microfluidic devices used for biofilm study [48] . With our device, we can precisely control the development of biofilm by intermittent flow of nutrients, completely isolate the biofilm from the media inlet and gradient-generating channels using the pneumatic valves, and sequentially introduce different cell types into the biofilm chamber. Of course, the ability to study a range of concentrations simultaneously with the eight channels (for example, Fig. 3c,d ) was instrumental in analysing the effect of various concentrations of 3 o C12HSL and IPTG. Bacterial QS systems have the attractive design features that they utilize diffusible signals [20] . Here we show, for the first time, that a QS system may be utilized with biofilm dispersal proteins to control consortial biofilm formation; that is, that an existing biofilm may be formed and then replaced by another biofilm, which then may be removed. These types of synthetic QS circuits may be used to pattern biofilms by facilitating the reuse of platforms and to create sophisticated reactor systems that will be used to form biorefineries. Although it may not be needed in practice to remove one biofilm with another, we chose to show this may be accomplished in order to show in principle that biofilms may be controlled; that is, that biofilms may be dispersed and that consortia populations may be controlled such that complex synthetic biocatalysis may be performed. Furthermore, these systems may be adopted in industrial and clinical processing as an alternative strategy to overcome the current limitations of biofilm control. Bacterial strains and growth conditions The bacterial strains and plasmids used in this study are listed in Supplementary Table S1 and were cultured at 37 °C. LB [49] with 0.2% glucose (LB-glucose) was used in all of the non-microfluidic experiments, and M9 [49] supplemented with 0.2% glucose (M9-glucose), LB-glucose, and tryptone medium (10 g of tryptone and 2.5 g of NaCl per litre) were used in the microfluidic device. Kanamycin (50 μg ml −1 ) was used for overnight cultures, chloramphenicol (100 μg ml −1 ) was used for maintaining the pCA24N-based plasmids and erythromycin (300 μg ml −1 ) was used for maintaining the pCM18-based plasmids. Plasmid construction All primers used for cloning are listed in Supplementary Table S2 . Plasmid pHha13D6 -gfp - lasI ( Fig. 2a ) contains hha13D6 (ref. 15 ) under the control of the IPTG-inducible T5-lac promoter, as well as gfp and lasI under the control of constitutive CP25 promoter. To form this plasmid, gfp was amplified by three rounds of PCR: the first PCR with primers gfp-F3 and gfp-R and template pCM18 (ref. 32 ) was to amplify gfp with the same RBS of rfp , and the second PCR with primers gfp-F2 and gfp-R using the first PCR product as a template, and the third PCR with primers gfp-F1 and gfp-R using the second PCR product as a template were performed to include the constitutive CP25 promoter of pCM18. pHha13D6- gfp was constructed by cloning the third PCR product into pCA24N- hha13D6 (ref. 15 ) using the NotI and BlpI restriction sites after hha13D6 sequence. The final construct pHha13D6- gfp - lasI was formed by cloning lasI with its native RBS from the P. aeruginosa PAO1 chromosome by using the lasI-F and lasI-R primers; the PCR product was cloned into pHha13D6- gfp using the BlpI restriction site. As a control plasmid for producing GFP and LasI but not producing Hha13D6, pGFP- lasI was constructed by inserting lasI into pCM18 using the lasI-F and lasI-R primers. Plasmid pBdcAE50Q -rfp - lasR ( Fig. 2b ) contains bdcAE50Q [16] under the control of the lasI promoter, as well as rfp and lasR under the control of the constitutive CP25 promoter. pBdcAE50Q was constructed by replacing the T5-lac promoter in pCA24N- bdcAE50Q [16] with the lasI promoter from P. aeruginosa using the plasI-F and plasI-R primers; the PCR fragment was cloned into the AvaI and BseRI restriction sites. Plasmid pDsRed- lasR was constructed by inserting lasR and its native RBS into the NotI site downstream of the rfp sequence in pDsRed-Express (Clontech) using the lasR-F and lasR-R primers. As a BlpI restriction site lies within lasR but was required for the next cloning steps, the BlpI site in pDsRed- lasR was disrupted by site-directed mutagenesis [15] (5′-GCTGAGC-3′ to 5′-TCTGAGC-3′) using the BlpIX-F and BlpIX-R primers (this mutation did not change the aa sequence), to form pDsRed-BlpIX- lasR . rfp and lasR were amplified from pDsRed-BlpIX- lasR by two rounds of PCR to include the constitutive CP25 promoter of pCM18: the first PCR was performed using the rfp-lasR-F2 and rfp-lasR-R primers, and the second PCR was performed using the rfp-lasR-F1 and rfp-lasR-R primers with the first PCR product. The final construct pBdcAE50Q- rfp - lasR was formed by inserting the rfp and lasR PCR products into the BlpI site downstream of bdcAE50Q in pBdcAE50Q. As a control plasmid for producing RFP and LasR but not producing BdcAE50Q, pRFP- lasR was constructed by inserting rfp and lasR using the rfp-lasR-F3 and rfp-lasR-R primers into pCM18-X, in which gfp was disrupted by introducing a truncation at Y66 of GFP using the gfpX-F and gfpX-R primers in pCM18. All plasmids were confirmed by PCR and DNA sequencing. Microfluidic device The poly(dimethyl)siloxane (PDMS)-based μBE device ( Fig. 1b ) was fabricated in the Materials Characterization Facility at Texas A&M University using conventional soft lithographic techniques [50] . The μBE device consists of a glass slide and two layers, a bottom layer, with a diffusive mixer and eight microchambers, and a top layer, which contains the pneumatic elements for controlling microvalves and a second diffusive mixer. The diffusive mixer in the bottom layer was used to generate different concentrations of dispersal signals (for example, IPTG for removing disperser cells) and to perfuse growth media into the biofilm microchambers. The mixer in the top layer was used to introduce bacteria into the microchambers at different cell densities ( Fig. 1b ). The dimensions of the diffusive mixers in both the top and bottom layers were 100 μm (width) ×150 μm (height) and 200 μm (width) ×200 μm (height), respectively, and the biofilm microchambers were 600 μm (width) ×150 μm (height). All pneumatic channels were 200 μm thick. The two layers were fabricated separately, and assembled by sequential oxygen plasma treatment and bonding (100 mTorr, 100 W, 40 s) in a reactive ion etcher. The top pneumatic layer was first aligned and bonded to the bottom diffusive mixer/microchamber membrane layer followed by bonding of the combined PDMS layer to a cover glass (22×50 mm). Tygon tubing (0.01′′ ID×0.03′′ OD, Saint Gobain performance plastics) was used for all fluidic connections. Two PicoPlus 11 syringe pumps (Harvard Apparatus) were used for each experiment to separately control fluid flow rates in the two layers. A temperature-controlled micro-incubator was used to maintain the temperature of the device at 37 °C. Moist air flowed continuously over the device in order to maintain humidity and avoid bubble formation inside the microchambers. The opening and closing of valves were pneumatically controlled by introducing vacuum or compressed air through the solenoid valves. The operation of solenoid valves and syringe pumps were remotely controlled through programs developed in-house for the LabVIEW platform (National Instruments). Microfluidic biofilm experiments For mono-species biofilm dispersal experiments, overnight cultures were washed and resuspended in M9 medium supplemented with glucose (0.2%) at a turbidity at 600 nm of ~1.0. The bacterial suspension was introduced into the eight biofilm microchambers through the top layer in the PDMS device ( Fig. 1b ). During this process, the main inlet valves ( Fig. 1b ) remained closed to prevent cells from entering and forming biofilm in the gradient-mixing channels, and to ensure proper mixing of dispersal signals before they enter the microchambers. The main outlet valves and seeding valves were then closed, and the culture was maintained without flow for 2 h to enable attachment of bacteria to the glass surface (seeding). After 2 h, both main inlet and outlet valves were opened, unattached cells were removed and the attached bacteria were allowed to grow by flowing LB-glucose at 2 μl min −1 . After 3 h, the medium was switched from LB-glucose to M9-glucose for 3 h because we found that a sudden depletion of nutrients promoted rapid development of biofilms. The biofilm was then developed for another 3 h by introducing LB-glucose into the chambers in a semi-batch mode (55-min static and 5-min flow). Thus, within 9 h after seeding, a robust and mature biofilm was formed. To disperse the biofilm, LB-glucose and LB-glucose containing a single concentration of the dispersal signal (IPTG for disperser cells and 3 o C12HSL for initial colonizer cells) was introduced through the two media inlets and allowed to mix in the serpentine gradient-generating channels to form eight concentrations of the dispersal signal in LB-glucose medium. Each stream leaving the diffusive mixer was used to perfuse a specific biofilm microchamber for 10 h. For dual-species biofilm dispersal experiments using 3 o C12HSL signalling, initial colonizer cell biofilms were developed uniformly across all eight microchambers for 9 h as for mono-species biofilms. During this 9-h period, unattached initial colonizer cells were continuously removed from the cell mixer and connecter tubing through the cell outlet by flowing M9 medium at 8 μl min −1 . After formation of the initial colonizer biofilm, disperser cells (turbidity at 600 nm of 2.0 in M9-glucose) were continuously perfused into the microchamber for 5 h to allow disperser cells to colonize the initial colonizer biofilm as well as the glass surface in vacant regions. After 5 h, LB-glucose was introduced into the microchamber in the semi-batch mode (55-min static and 5-min flow) for 28–30 h. The static condition ensured biofilm development and build-up of 3 o C12HSL needed for induction of the BdcAE50Q dispersal protein in initial colonizer cells. To remove the disperser cell biofilm, LB-glucose containing 2mM IPTG was introduced in semi-batch mode for 18 to 20 h. For dual-species biofilm dispersal experiments using arabinose, initial colonizer cell biofilms were developed as a gradient across the eight microchambers for 10 h, then a uniform concentration of disperser cells were seeded for 5 h in all eight channels in LB-glucose medium. After 21 h, 1% arabinose in tryptone medium was added for an additional 26 h to disperse the initial colonizer biofilm. How to cite this article: Hong, S.H. et al . Synthetic quorum-sensing circuit to control consortial biofilm formation and dispersal in a microfluidic device. Nat. Commun. 3:613 doi: 10.1038/ncomms1616 (2012).